Synthesis of luminescent europium defects in diamond Lanthanides are vital components in lighting, imaging technologies and future quantum memory applications owing to their narrow optical transitions and long spin coherence times. Recently, diamond has become a pre-eminent platform for the realisation of many experiments in quantum information science. Here we demonstrate a promising approach to incorporate Eu ions into diamond, providing a means to harness the exceptional characteristics of both lanthanides and diamond in a single material. Polyelectrolytes are used to electrostatically assemble Eu(III) chelate molecules on diamond and subsequently chemical vapour deposition is employed for the diamond growth. Fluorescence measurements show that the Eu atoms retain the characteristic optical signature of Eu(III) upon incorporation into the diamond lattice. Computational modelling supports the experimental findings, corroborating that Eu(III) in diamond is a stable configuration. The formed defects demonstrate the outstanding chemical control over the incorporation of impurities into diamond enabled by the electrostatic assembly together with chemical vapour deposition growth. Rare earth ions are vital components of many modern technologies including lasers, light emitting diodes and communications [1] , [2] , [3] , [4] , [5] . The storage of quantum bits is critical to future quantum information technologies. Lanthanides exhibit remarkably long nuclear spin coherence times; europium exhibits nuclear spin coherence times that are extremely long (T 2 -minutes T 1 -weeks), making it a superb candidate for such quantum memories or for applications in magnetic sensing [6] , [7] , [8] . In addition, Eu(III) has drawn attention for its photostable, narrowband fluorescence lines across in the visible. Coherent manipulation of several spin-selective transitions allows optical detection of the nuclear spin state enabling their implementation as local NMR probes [9] , [10] , [11] . Currently, diamond is one of the pre-eminent platforms for high resolution magnetometry and quantum information processing, owing to the nitrogen vacancy (NV) defect [12] , [13] , [14] , [15] . Diamond possesses a very large band gap (5.5 eV) that can accommodate a variety of optically active defects. Furthermore, the progress in growing isotopically pure diamond, (by minimising 13 C isotopes) has recently enabled very long spin coherence times of the NV [16] , [17] . The chemical stability of diamond means that nanodiamonds exhibit excellent photostability and cytotoxicity—making them promising as bio-labels and biosensors. Combining the extreme properties of diamond with the unique atomic and optical properties of rare earth ions is an important first step towards an all diamond solid state platform for quantum information processing and sensing. In this work we demonstrate computationally that Eu is stable within the diamond matrix and show that the native f-orbital transitions of a Eu(III) atom should be preserved. We then present a robust method to incorporate Eu ions into diamond using chemical self assembly and growth. A layer-by-layer approach is employed to first electrostatically assemble a positively charged polymer on an oxidised diamond surface and then assemble a negatively charged Eu complex on top of the polymer. The coated diamond is then transferred into a chemical vapour deposition chamber for a subsequent overgrowth of diamond to generate a Eu-doped layer. This technique has the advantage that nearly any atomic species that can be electrostatically assembled on the diamond surface can be incorporated in diamond. Currently ion implantation is commonly used to dope solids with external ions, however this approach can irreversibly damage the host matrix. In the technique presented in this work, the doping process occurs using a bottom-up method that does not damage the host matrix and preserves the atomic transitions of the alien atom. Simulations To understand the feasibility of incorporating lanthanide defects into the diamond lattice, the energetics of a Eu defect within the diamond lattice was simulated. The formation energy is calculated for Eu in diamond using density functional theory within the local spin density approximation as implemented in the WIEN2K code [18] . A 64-site supercell is considered, corresponding to a cube of 2 × 2 × 2 nonprimitive cubic unit cells of diamond, with a europium atom substituted in the centre and next to 1, 2 or 3 carbon vacancies. There is insufficient space in the crystal lattice for Eu to substitute for C without any vacancies. A k-point mesh of 4 × 4 × 4 is used to sample the irreducible Brillouin zone. The Coulomb interaction parameter U and exchange parameter J are set to 7.397 eV and 1.109 eV, respectively, and the spin-orbit interaction is neglected [19] . 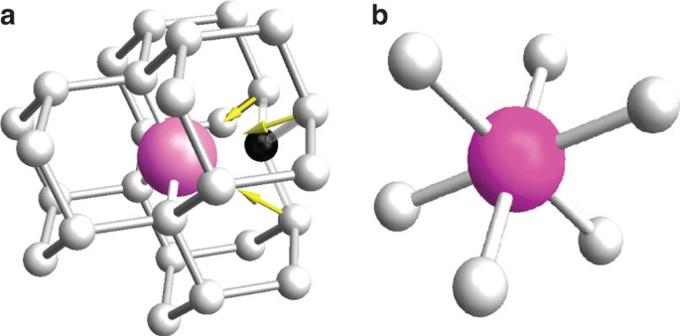Figure 1: The relaxation process in one vacancy structure. (a) After the substitution of Eu, three nearest neighbor carbons of europium and another three carbons bonded with the taken carbon will relax towards the Eu. (b) A defect center with a sixfold coordinate shell of carbon atoms will be formed after relaxation. The formation energy and 4f-shell occupation for charge states of Eu ranging from −2 to +4 have been calculated for a Fermi energy at the top of the valence band, and are shown in Table 1 . The top of the valence band provides a reference point for these formation energies. It is then possible to use our calculations to determine the formation energy for the defect if the Fermi energy were located somewhere in the middle of the gap. Note that the 4f occupation is almost entirely independent of the charge state of the defect. Table 1 Formation energy and 4f electron occupation of the Eu defect. Full size table It is known that correlation effects in the 4f series stabilise the f-shell occupation relative to 5s and 5p occupation [20] , even as the charge state of the ion varies for 4f levels in the band gap. Hence we find that the average 4f occupation remains relatively stable (near that expected for the +3 state of the isolated atom) even as the actual defect charge state varies from −2 to +4. A single vacancy is found to be the most stable configuration with Eu; in the relaxed positions of the atoms the carbon neighbours of the vacancy relax towards the Eu, forming a sixfold coordinated shell of carbon atoms surrounding the Eu, as shown in Fig. 1 . Figure 1: The relaxation process in one vacancy structure. ( a ) After the substitution of Eu, three nearest neighbor carbons of europium and another three carbons bonded with the taken carbon will relax towards the Eu. ( b ) A defect center with a sixfold coordinate shell of carbon atoms will be formed after relaxation. Full size image Experimental synthesis In preliminary studies we were unable to create luminescent europium defects via ion implantation of Eu into the diamond crystal. Even after annealing at 1,000 °C no signature of the Eu complexes was observed [21] . To eliminate the implantation-related damage, a technique was developed to introduce Eu into the diamond matrix during microwave chemical vapour deposition growth. The process used to prepare a diamond having a monolayer of Eu for growth is shown in Fig. 2 . 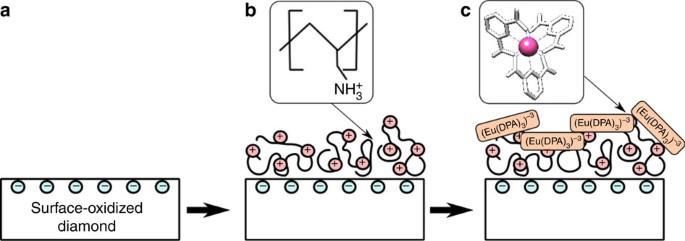Figure 2: An overview of the process used to assemble the Eu precursor on a bulk diamond before growth. (a) The surface of the diamond is oxidized using a boiling tri-acid etch, (b) A positively charged polymer, PAH, is assembled electrostatically on the negatively charged diamond (c) The Eu precursor, [Eu(III) tridipicolinate]−3is assembled on the positively charged polymer. Figure 2: An overview of the process used to assemble the Eu precursor on a bulk diamond before growth. ( a ) The surface of the diamond is oxidized using a boiling tri-acid etch, ( b ) A positively charged polymer, PAH, is assembled electrostatically on the negatively charged diamond ( c ) The Eu precursor, [Eu(III) tridipicolinate] −3 is assembled on the positively charged polymer. Full size image A monolayer was desired to minimise the impact of the Eu on the growth conditions. To assemble this monolayer, first the diamond was surface oxidised using a boiling tri-acid etch (1:1:1 nitric:sulphuric:perchloric acids) to create a negatively charged surface. Next, polyallylamine hydrochloride (PAH), a positively charged polymer, was assembled on the negatively charged diamond surface. Finally, a negatively charged europium complex, Eu(III) tri-(2,6-pyridine dicarboxylic acid) (EuDPA), was assembled on the positively charged polymer layer. The use of a chelated Eu complex and the polymer layer may seem superfluous, however they are both critical to the assembly of an Eu(III) monolayer on the diamond. The surface of oxidised diamond is significantly negatively charged at above pH 5. Unfortunately, at elevated pH Eu(III) rapidly forms oxides and hydroxides and precipitates out of the solution. Eu oxides are stable even at the elevated temperatures present during chemical vapour deposition diamond growth, making them nonideal for the facile incorporation of Eu into diamond. Three different techniques were used to prepare Eu:nanodiamond substrates for growth: (1) 5 nm nanodiamond seeds were mixed with an aqueous solution of EuDPA and deposited on SiO 2 on Si; (2) nanodiamonds were oxidised in boiling acid, coated with PAH and then coated with EuDPA and then deposited on SiO 2 on Si; (3) the SiO 2 substrate was treated with hot piranha to create a highly negatively charged surface, then PAH was assembled on the substrate followed by the assembly of EuDPA and lastly nanodiamonds were dispersed on the coated substrate. The diamond growth was carried out in a conventional microwave-assisted chemical vapour deposition reactor under pressure of 60 torr and 900 W microwave plasma. The duration of the growth was ~10 min to grow individual nanodiamonds. Post-growth the diamond specimens were characterised by photoluminesence spectroscopy. Samples were excited with a 395 nm-pulsed laser. The fluorescence for a bulk diamond sample containing Eu is shown in Fig. 3a . The fluorescence of the Eu in diamond (3a, bottom, blue curve) differs from that of the precursor (3a, top, red curve). The strongest peak, corresponding to the 5 D 0 → 7 F 2 transition, is a singlet in the precursor and a multiplet in the diamond sample. The 5 D 0 → 7 F 1 and 5 D 0 → 7 F 4 transitions are significantly broadened, perhaps also as a result of peak splitting. Lastly, the Eu in diamond exhibits an additional singlet at 582 nm that is not present in the precursor, likely corresponding to the 5 D 0 → 7 F 0 transition. 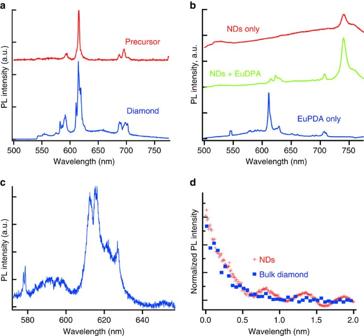Figure 3: Ensemble Photoluminescence measurements of europium defects. (a) PL from the EuDPA precursor (top) and Eu defects in bulk diamond after growth (bottom). (b) PL of nanodiamonds grown without Eu (top), nanodiamonds grown with EuDPA (middle) and EuDPA grown without nanodiamonds (bottom). (c) A high resolution PL spectrum of the Eu defect in nanodiamonds revealing the line splitting of the5D0→7F1transition. (d) Fluorescence decay of Eu defects in bulk diamond (blue squares) and nanodiamonds (red cross). Figure 3: Ensemble Photoluminescence measurements of europium defects. ( a ) PL from the EuDPA precursor (top) and Eu defects in bulk diamond after growth (bottom). ( b ) PL of nanodiamonds grown without Eu (top), nanodiamonds grown with EuDPA (middle) and EuDPA grown without nanodiamonds (bottom). ( c ) A high resolution PL spectrum of the Eu defect in nanodiamonds revealing the line splitting of the 5 D 0 → 7 F 1 transition. ( d ) Fluorescence decay of Eu defects in bulk diamond (blue squares) and nanodiamonds (red cross). Full size image Photoluminescence measurements of nanodiamonds grown via each technique showed that all three techniques lead to Eu defects in the nanodiamond. However, simply mixing the Eu complex with the nanodiamonds (technique 1) led to the formation of large unknown crystallites that produce a broad background fluorescence signal while the Eu-associated fluorescence signal was significantly weaker for the nanodiamonds that were coated with Eu (technique 2), perhaps because of less total Eu available during growth. The third technique proved most effective. A fluorescence spectrum of Eu nanodiamonds is shown in Fig. 3b (middle). Spectra of nanodiamonds grown without the Eu precursor (3b top) and a sample with the Eu precursor but no nanodiamond seeds (3b bottom) are shown for comparison. The spectrum for the Eu nanodiamonds is distinctly different for that of the precursor grown without any seeds. The peak at 738 nm seen in the samples grown with a nanodiamond seed (3b top and middle) is characteristic of silicon vacancies (SiV) in diamond, likely introduced owing to the Si substrate on which the nanodiamonds were grown [22] . A higher resolution spectrum of the 5 D 0 → 7 F 2 transition for the nanodiamond sample is shown in Fig. 3c , detailing the splitting of this peak. The splitting of the fluorescence transitions for Eu(III) in diamond suggests that the symmetry of the local environment around the Eu is lower than the symmetry of an isolated Eu atom. Calculations show that the environment for Eu will be a locally distorted (and strained) environment, for the atomic relaxations associated with Eu-V (or more vacancy) complexes are substantial. Furthermore, with many Eu-#V complexes of similar formation energies, it is likely that Eu appears with a variable number of vacancies, leading to broadening of the line. The lower symmetry associated with the Eu and vacancies may introduce nonradiative pathways, however the radiative emission is clearly seen from the Eu dopants so the photoluminescence is not entirely quenched. To fully understand the precise splitting of the Eu(III) transitions detailed analysis of the symmetry of the defect centre in relation to the crystal field is required. Fluorescence lifetime measurements, shown in Fig. 3d were recorded from both the Eu bulk and Eu nanodiamond samples. The Eu defect in the nanodiamond sample exhibited a lifetime of 325 μs while the lifetime of the defects in the bulk sample were slightly longer, 391 μs. Remarkably, however, the measured lifetime of the Eu defects in diamond is shorter than other reported Eu-related complexes [8] , [23] . The short lifetime may be attributed to the wide band gap of the diamond lattice, which localises the wave functions of the 4f levels strongly and thus enhances the emission. Alternatively, one may consider potential quenching mechanisms owing to a strained environment that may provide nonradiative pathways. Nevertheless, the radiative emission is clearly seen from the Eu defect. The nanodiamonds are smaller than the diffraction limit of light, so to further verify that the Eu(III) fluorescence was indeed associated with individual nanodiamonds, cathodoluminescence (CL) studies of single nanodiamonds using 10 keV electron beam were carried out in situ within a scanning electron microscope (SEM). The light is collected using a parabolic mirror and directed into a spectrometer. Fig. 4a shows a SEM image of several individual nanodiamonds that were grown on top of the Eu-containing polymer. Fig. 4b shows the recorded CL signal unveiling the common A band at 460 nm (attributed to nitrogen aggregates in diamond), the narrow peak at 738 nm [24] , attributed to the SiV and the emission centred at 612 nm, associated with a Eu complex in diamond. Interesting to note, that even in CL measurements the Eu signal in diamond is replicated, indicating the possible transition pathways from the excited state to the Eu levels. Owing the complex electron beam dynamics, not all colour centres are visible in CL. The availability of imaging Eu defects with CL opens important possibilities for detailed characterisation of these defects using time-resolved high resolution CL methods. The nanodiamond specimens characterised by CL were grown using the third technique. In this synthesis the entire precursor was destroyed and Eu was consumed or dissipated during growth and consequently no background Eu fluorescence was observed from the regions between nanodiamonds. 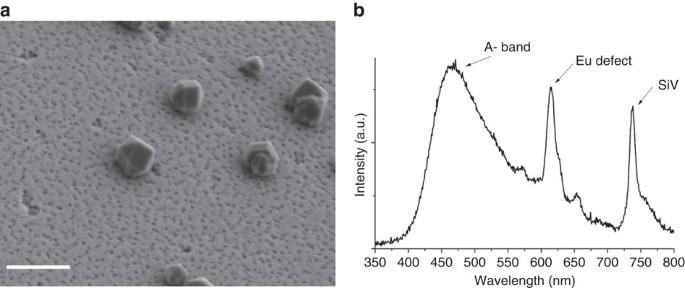Figure 4: CL imaging of Eu defects in nanodiamonds. (a) SEM image of the nanodiamonds containing Eu defects, employing the technique #3. Scale bar, 500 nm (b) CL signal recorded from an individual nanodiamonds, resolving the A band fluorescence (broad emission at ~460 nm), the SiV defect (~738 nm) and the Eu line (~612 nm). Figure 4: CL imaging of Eu defects in nanodiamonds. ( a ) SEM image of the nanodiamonds containing Eu defects, employing the technique #3. Scale bar, 500 nm ( b ) CL signal recorded from an individual nanodiamonds, resolving the A band fluorescence (broad emission at ~460 nm), the SiV defect (~738 nm) and the Eu line (~612 nm). Full size image Formation of other defects in diamond using the self assembly electrostatic technique To demonstrate the broad utility of this technique for creating colour centres in diamond, chromate was electrostatically assembled on the surface of a bulk diamond, as described for the EuDPA complex above. Chromate was selected because chromium-activated centres exhibit fluorescence that is distinct from the native ion. After growth, photoluminescence measurements, revealed a very sharp resonance centred at 761.14 nm, as shown in Fig. 5 , in accordance to the previous results on chromium-related colour centres in diamond [25] , [26] , [27] . Therefore, the chemical technique is a viable rote for engineering colour centres in diamond and potentially other wide band gap semiconductors. 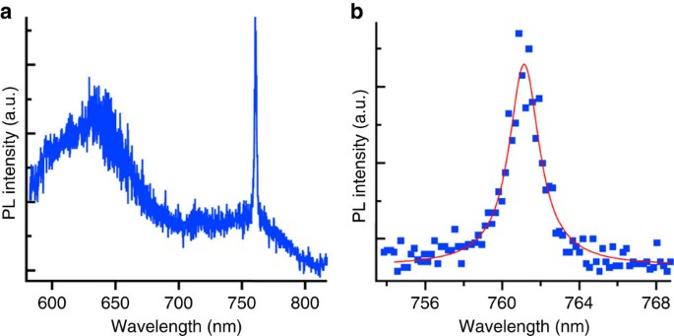Figure 5: Optical properties of chromium-activated defects in diamond created by electrostatically assembling chromate on a bulk diamond. (a) PL spectrum from the Cr related defect. (b) A magnification of the sharp Cr-defect resonance. Figure 5: Optical properties of chromium-activated defects in diamond created by electrostatically assembling chromate on a bulk diamond. ( a ) PL spectrum from the Cr related defect. ( b ) A magnification of the sharp Cr-defect resonance. Full size image The incorporation efficiency of the Eu atoms into the growing diamond crystals is sufficiently high. Most of the nanocrystals showed the Eu signal and the incorporation of the Eu in a bulk was homogeneous across the sample with no preferred agglomeration. Given that the fluorescence lifetime is long (~300 μs) and the observed fluorescence is at the same order as the emission from the SiV (that has only ~2 ns lifetime) we conclude that the concentration of the Eu is at the p.p.m. level. To incorporate the Eu atoms at a single defect level, it is possible to dramatically reduce the growth speed and dilute the Eu precursor. However, as the fluorescence lifetime is considerably long, it would be hard to detect over the background noise using conventional confocal microscopy. We presented a chemical method to engineer Eu-related defects in diamond. The incorporation of Eu into diamond while retaining the optical transitions associated with Eu(III) is an important first step towards developing an all diamond platform for quantum memory [28] or computation. Further measurement of the spin properties of the embedded Eu defects are needed to fully exploit the potential of this system. Since the process involves the introduction of the Eu during growth there is no residual damage to the diamond lattice as is caused via ion implantation. Finally, this versatile method can be extended to many other atomic species including other lanthanides such as Pr and Gd that may be of particular interest given the unique optical and magnetic properties of these species. Preparation of Eu(III) tri(2,6-pyridine dicarboxylic acid) Dipicolinic acid (DPA) (0.5 g, Sigma Aldrich) was dissolved in 10 ml of water. NaOH (3.3 ml, 2 M) was added to DPA solution to deprotonate the acid. The solution was brought to a boil while stirring magnetically until the DPA was dissolved. A solution of EuCl 3 ·6H 2 O (0.267 g in 1 ml) was added to the DPA solution. The solution was allowed to cool and 0.2 M NaOH was added dropwise until the solution reached a pH of 8. Addition of NaOH too rapidly will lead to the irreversible formation of a white precipitate of europium oxide or hydroxide. The solution was left in a fume hood to crystalize and yellow EuDPA crystals were removed from the mother liquor, and were rinsed and dried. Deposition of EuDPA on bulk diamond A 3 × 3 mm diamond (Element Six) was cleaned in boiling tri-acid (1:1:1 HNO 3 :HClO 4 :H 2 SO 4 , 133 μl each). The solution was heated in a sand bath to ~300 °C in small round bottom flask with condenser. The diamond was left to sit for 1 h and the heat was turned off. The diamond was allowed to cool overnight in the acid solution and rinsed 3 × in ultrapure water. The diamond was incubated overnight in a solution of PAH (50k MW, 0.1 M by monomer, Sigma Aldrich) adjusted to pH 8.0. A pH of 8.0 or higher is critical for having a negatively charged diamond surface. Excess PAH was rinsed off with ultrapure water. To coat with EuDPA, the PAH-treated diamond was incubated for 3 h with a 0.1 M solution of EuDPA adjusted to pH 3.8. The diamond was incubated for 3 h and rinsed thoroughly. Co-deposition of EuDPA and nanodiamonds A dilute solution (1 mg ml −1 ) of seed nanodiamonds (1 ml, 4–6 nm) was centrifuged (10,000 r.p.m., 15 min) to form a pellet. The nanodiamond pellet was rinsed 3 × with ultrapure water and then resuspended in about 1 ml of the same. A 50 μl aliquot of the solution of cleaned nanodiamonds was co deposited with 50 μl of EuDPA solution (10 mg ml −1 , no pH adjustment) on a cleaned 1 cm square piece of a polished Si wafer. After growth under conditions described in the main manuscript the unknown crystallites were observed together with the nanodiamonds as shown in Fig. 6 . The unknown crystallites are several microns in size and induce broad background fluorescence. They can be easily separated by ultrasonication and rinsing of the substrate after growth. 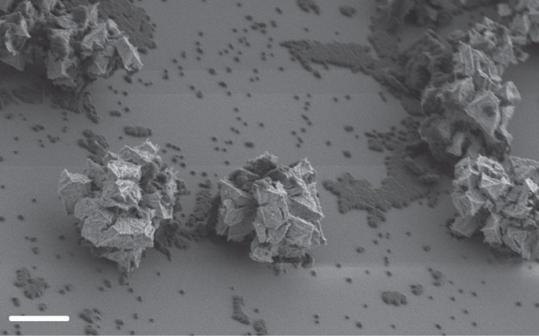Figure 6: SEM image of the unknown crystallites. Scale bar, 5 μm. Figure 6: SEM image of the unknown crystallites. Scale bar, 5 μm. Full size image Coating nanodiamonds with EuDPA Nanodiamonds (500–1,000 nm) were oxidised in boiling tri-acid (as described for bulk diamond) for 6 h and allowed to cool fully. The solution of nanodiamonds and tri-acid was carefully centrifuged and the acid solution was removed. The nanodiamonds were then rinsed thoroughly with ultrapure water to remove residual acid. The nanodiamonds were then resuspended at a concentration of 10 mg ml −1 in an aqueous solution of PAH (50k MW, 0.1 M by monomer, adjusted to pH 8.0). The PAH-coated nanodiamonds were centrifuged to form a pellet, rinsed with ultrapure water and repelleted. The pellet of PAH-coated nanodiamonds was resuspended in 10 mg ml −1 EuDPA (1 ml) and incubated overnight. The coated nanodiamonds were again rinsed with ultrapure water and deposited on a piece of Si for growth. Depositing Eu on SiO 2 A 1 cm square piece of thermally grown SiO 2 on Si was oxidised in a hot piranha bath. The substrate was incubated with an aqueous solution of PAH (0.1 M by monomer, adjusted to pH 8) for 1 h. The substrate was rinsed with copious ultrapure water to remove unbound polymer and then incubated with a solution of EuDPA (10 mg ml −1 , pH 3.9) for 1 h. The sample was again rinsed with ultrapure water to remove excess EuDPA. Before growth 4–6 nm nanodiamond seeds were deposited on the substrate. Coating bulk diamond with chromate A 3 × 3 mm bulk diamond was oxidised via tri-acid etch (described above). The specimen was rocked in 1 ml of PAH solution (0.2 M, adjusted to pH 8.0 w/1 M NaOH) overnight. The specimen was rinsed thoroughly with ultrapure water. The PAH-coated diamond was incubated with 1 ml of aqueous solution of potassium chromate (0.1 M, adjusted to pH 5) for 3 h and then rinsed thoroughly with ultrapure water. Diamond growth The diamond growth was carried out in a conventional microwave-assisted chemical vapour deposition reactor (Seki Technotron, Model: AX5010-INT) under pressure of 60 torr and 900 W microwave plasma. The methane to hydrogen flow ratio was 4:400 standard cubic centimetre per minute. No heating stage was used during the growth. The single crystal growth was ~10 min to achieve~200 nm thick overgrown crystal. Optical measurements Ensemble photoluminescence measurements were performed at room temperature using a frequency-doubled titanium sapphire laser (Mira 900), emitting at 395 nm. The excitation was passed through a dichroic mirror onto a high (0.9) numerical aperture objective (Nikon). The light was collected through the same objective and directed onto a spectrometer. Confocal scanning was achieved using a 2D scanning piezo stage (Thorlabs). How to cite this article: Magyar, A. et al. Synthesis of luminescent europium defects in diamond. Nat. Commun. 5:3523 doi: 10.1038/ncomms4523 (2014).